PPARγ contributes to PKM2 and HK2 expression in fatty liver Rapidly proliferating cells promote glycolysis in aerobic conditions, to increase growth rate. Expression of specific glycolytic enzymes, namely pyruvate kinase M2 and hexokinase 2, concurs to this metabolic adaptation, as their kinetics and intracellular localization favour biosynthetic processes required for cell proliferation. Intracellular factors regulating their selective expression remain largely unknown. Here we show that the peroxisome proliferator-activated receptor gamma transcription factor and nuclear hormone receptor contributes to selective pyruvate kinase M2 and hexokinase 2 gene expression in PTEN -null fatty liver. Peroxisome proliferator-activated receptor gamma expression, liver steatosis, shift to aerobic glycolysis and tumorigenesis are under the control of the Akt2 kinase in PTEN -null mouse livers. Peroxisome proliferator-activated receptor gamma binds to hexokinase 2 and pyruvate kinase M promoters to activate transcription. In vivo rescue of peroxisome proliferator-activated receptor gamma activity causes liver steatosis, hypertrophy and hyperplasia. Our data suggest that therapies with the insulin-sensitizing agents and peroxisome proliferator-activated receptor gamma agonists, thiazolidinediones, may have opposite outcomes depending on the nutritional or genetic origins of liver steatosis. Glycolysis generates energy and intermediates for macromolecule biosynthesis. Hence the growth factors, anabolic hormones and oncogenic events perfected molecular mechanisms to upregulate glycolytic enzyme activities and gene expression [1] . The phosphatidylinositol-3-kinase (PI3K) pathway, a master regulator of cell growth, proliferation and metabolism in response to insulin, growth factors and oncogenic insults, is a potent stimulator of glycolysis by acting on different levels, from the upregulation of glucose uptake at the membrane, to the post-translational modifications of glycolytic enzymes, to the induction of glycolytic gene expression [2] . In the nucleus, the transcription factor c-Myc, encoded by the MYC oncogene, directly binds and activates the majority of glycolytic gene promoters [3] . In addition, the hypoxia-inducible factor 1 (HIF-1), which can accumulate in cells as a consequence of inactivating mutations in the Von Hippel–Lindau ( VHL ) tumour suppressor gene, cooperates with c-Myc on the transcriptional activity of the glycolytic gene promoters [4] . Further complexity comes from the existence of multiple isozymes catalysing specific reactions in glycolysis. For instance, four hexokinases (HK1-4) catalyse the first step of glycolysis, that is, the phosphorylation of glucose, while four pyruvate kinases (PKM1, PKM2, PKL, PKR) catalyse the last step of glycolysis, that is, the final conversion of phosphoenolpyruvate to pyruvate. These isozymes display differential tissue distribution and confer specific kinetic and regulatory properties to the glycolytic flux [5] , [6] , [7] . However the molecular mechanisms favouring selective expression of specific isozymes remain mysterious. Pyruvate, the end product of glycolysis, can be reduced to lactate in the cytosol during anaerobic conditions or enter the mitochondria to be further oxidized during aerobic respiration. In rapidly dividing cells, lactate production is also observed under normal oxygen conditions, a phenomenon called aerobic glycolysis or Warburg effect, which may provide a growth advantage by producing carbon intermediates as building blocks for cellular components [1] . Among the glycolytic isozymes, the expression of hexokinase 2 (HK2) and the M2 isoform of pyruvate kinase (PKM2) may particularly favour aerobic glycolysis and cell proliferation owing to their intracellular localization and kinetic properties. The features of HK2 that may favour aerobic glycolysis are mitochondrial localization that allows the consumption of mitochondrially produced ATP to start glycolysis, a relatively high affinity for glucose and presence of two catalytically active domains that double the rate of glucose-6-phosphate formation [5] , [6] . Although the other pyruvate kinase isozymes are exclusively tetrameric enzymes, PKM2 can also switch to a less active dimeric form by allosteric regulation in presence of mitogenic signals, leading to the accumulation of glycolytic intermediates that can be used to increase the biomass [8] . Consistently, HK2 and PKM2 isozymes are reported to be predominantly expressed in highly malignant tumours, and their functional role in promoting tumour progression has been demonstrated [7] , [9] . Particularly, a relative switch from HK4 (also named glucokinase) to HK2, and from PKL to PKM2 has been observed during progressive stages of liver transformation [10] , [11] , [12] . In liver, insulin signalling through the PI3K pathway has a fundamental role in the regulation of lipid and glucose metabolism, and pathophysiological growth. Gene deletions abrogating PI3K activity in mouse liver lead to severe insulin resistance, glucose intolerance, increased glucose output and defective lipid neogenesis [13] . Conversely, mutations activating the PI3K pathway, including the liver-specific deletion of the phosphatidylinositol (3,4,5)-triphosphate-lipid phosphatase and tumor suppressor PTEN (phosphatase and tensin homologue) gene, caused insulin hypersensitivity, improved glucose tolerance, hepatomegaly, steatosis in young adult mice, followed by adenocarcinoma formation since 7 months of age [14] , [15] . Among the PI3K-dependent effectors, the serine/threonine kinase Akt2 is required for the regulation of hepatic glucose output, lipid accumulation, and tumorigenesis in PTEN -null livers [16] , [17] , [18] , [19] . In this report, we therefore performed genetic epistasis experiments to address the impact of PI3K/Akt2 activity on liver glycolysis. Strikingly, we find that, whereas PTEN deletion causes a general upregulation of glycolytic gene expression, Akt2 selectively controls HK2 and PKM2 isozymes. We identify peroxisome proliferator-activated receptor gamma (PPARγ) nuclear hormone receptor as a novel transcription factor turning on these specific glycolytic isozymes that are frequently upregulated in pathophysiological growth. Activation of glycolysis in PTEN -null liver Consistent with the positive role of the PI3K pathway on the cell switch to glycolytic metabolism [2] , PTEN -null mouse livers showed a global upregulation of glycolytic enzymes ( Fig. 1 ). The expression of multiple glycolytic enzymes that are commonly expressed in liver, including glucokinase (GCK), glucose phosphate isomerase 1 (GPI1), glyceraldehyde 3-phosphate dehydrogenase (GAPDH), enolase 1 (ENO1), phosphoglycerate kinase 1 (PGK1) and L-type pyruvate kinase (PKL) was augmented at the messenger RNA and protein levels ( Fig. 1a,b ). The increase in expression paralleled increased enzymatic activity, while mitochondrial enzymes such as citrate synthase and cytochrome c oxydase were not affected ( Supplementary Fig. S1 ). These metabolic changes were concomitant with liver triglyceride accumulation (steatosis) and hyperplasia, hypoglycaemia and insulin hypersensitivity, and preceded the adenocarcinoma formation that was observed since 7 months of age [14] , [15] ( Supplementary Fig. S2 ). As Akt2 has a crucial role mediating the action of insulin and PI3K on hepatic glucose homeostasis, steatosis, hyperplasia and tumorigenesis [16] , [17] , [19] ( Supplementary Fig. S2 ), we addressed the effect of Akt2 deletion on glycolysis of PTEN -null livers. Surprisingly, the upregulation of all the above mentioned glycolytic enzymes was also observed in AlbCre;PTEN f/f ;Akt2 −/− livers ( Fig. 1a,b ; Supplementary Fig. S1 ), ruling out an involvement of Akt2 in this general activation of glycolysis. 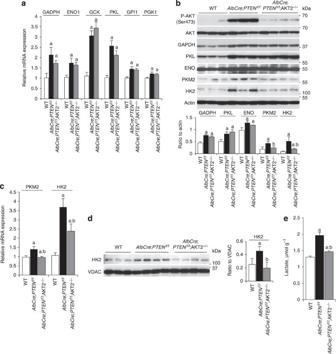Figure 1: Akt2 controls expression of specific glycolytic isozymes inPTEN-null liver. Relative transcript (a) and protein (b) levels of glycolytic enzymes in the mouse livers of indicated genotypes. For protein analysis, the ratio to β-actin of the densitometric assay is presented. Data are mean±s.e.m.,n=3–7 (P<0.05 (a) versus WT; (b) versusAlbCre;PTENf/f; 2-tailed, unpaired Student'sttest). (c) RT–QPCR for PKM2 and HK2 expression from mice livers of indicated genotypes. Data are mean ±s.e.m.,n=7 (P<0.05 (a) versus WT; (b) versusAlbCre;PTENf/f; 2-tailed, unpaired Student'sttest). (d) Immunoblot analysis of HK2 in liver mitochondria extracts from mice of indicated genotypes. The ratio to VDAC of the densitometric assay ±s.e.m. is presented,n=3–4 (P<0.05 (a) versus WT; (b) versusAlbCre;PTENf/f; 2-tailed, unpaired Student'sttest). (e) Hepatic lactate levels of random-fed mice of indicated genotypes. Data are mean ±s.e.m.,n=5–8 (P<0.05 (a) versus WT; (b) versusAlbCre;PTENf/f; 2-tailed, unpaired Student'sttest). Figure 1: Akt2 controls expression of specific glycolytic isozymes in PTEN -null liver. Relative transcript ( a ) and protein ( b ) levels of glycolytic enzymes in the mouse livers of indicated genotypes. For protein analysis, the ratio to β-actin of the densitometric assay is presented. Data are mean±s.e.m., n =3–7 ( P <0.05 (a) versus WT; (b) versus AlbCre;PTEN f/f ; 2-tailed, unpaired Student's t test). ( c ) RT–QPCR for PKM2 and HK2 expression from mice livers of indicated genotypes. Data are mean ±s.e.m., n =7 ( P <0.05 (a) versus WT; (b) versus AlbCre;PTEN f/f ; 2-tailed, unpaired Student's t test). ( d ) Immunoblot analysis of HK2 in liver mitochondria extracts from mice of indicated genotypes. The ratio to VDAC of the densitometric assay ±s.e.m. is presented, n =3–4 ( P <0.05 (a) versus WT; (b) versus AlbCre;PTEN f/f ; 2-tailed, unpaired Student's t test). ( e ) Hepatic lactate levels of random-fed mice of indicated genotypes. Data are mean ±s.e.m., n =5–8 ( P <0.05 (a) versus WT; (b) versus AlbCre;PTEN f/f ; 2-tailed, unpaired Student's t test). Full size image Akt2 controls expression of HK2 and PKM2 in PTEN -null liver Specific glycolytic isozymes, namely HK2 and PKM2 have been demonstrated to favour aerobic glycolysis and growth [7] , [20] . PKM2 and HK2 are expressed at low levels in wild-type adult mouse livers. As shown in Figure 1b and in Figure 1c , PTEN deletion upregulated HK2 and PKM2 mRNA and protein expression. Importantly, Akt2 deletion was sufficient to reduce by 40–60% the expression of both isozymes at 3 months of age, well before tumour onset. In addition, Akt2 deletion also blunted mitochondrial levels of HK2 ( Fig. 1d ), which should affect ATP usage towards glycolysis [20] . Finally, the difference in HK2 and PKM2 expression in AlbCre;PTEN f/f ;Akt2 −/− livers was accompanied by lower levels of hepatic lactate as compared with AlbCre;PTEN f/f ( Fig. 1e ). Taken together, these data indicate that Akt2 promotes aerobic glycolysis in PTEN -null fatty liver. Expression of HK2 and PKM2 isozymes promotes liver growth To evaluate the functional outcome of glycolytic isozymes expression on liver pathophysiology, adenoviral-mediated HK2 overexpression was achieved in vivo ( Fig. 2a ). HK2 overexpression led to a 100% increase in liver mass in wild type, and a 135% increase in AlbCre;PTEN f/f ;Akt2 −/− mice ( Fig. 2b ). In addition, HK2 promoted lactate production, steatosis and hepatocyte proliferation ( Fig. 2c,d,e ). HK2 also upregulated triglyceride content and lactate release after 60 h of overexpression in wild-type primary hepatocyte cultures ( Supplementary Fig. S3 ). PKM2 overexpression in vivo in wild-type mice caused a 74% increase in liver mass, an effect that was comparable to HK2 ( Fig. 2b ). The combination of both HK2 and PKM2 further increased liver mass to 134% as compared with green fluorescent protein (GFP)-treated control mice. Thus HK2 and PKM2 overexpression at supraphysiological levels is sufficient to cause liver steatosis and growth. In conclusion, a specific pattern of glycolytic isozyme expression correlates with the Akt2-dependent steatosis, hyperplasia and oncogenic potential of PTEN -null liver cells. 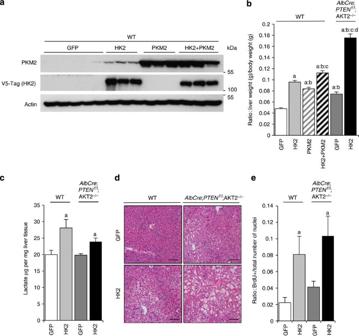Figure 2: HK2 and PKM2 glycolytic isozyme expression promotes liver growth. (a) Immunoblot analysis of PKM2 and HK2 protein expression in livers of mice, 7 days after transduction with indicated adenoviruses. (b) Liver weight relative to body weight of mice transduced with indicated adenoviruses. Data are means±s.e.m.,n=3–8 (P<0.05 (a) versus GFP/WT; (b) versus adenoHK2/WT; (c) versus adenoPKM2/WT; (d) versus GFP/AlbCre;PTENf/f;Akt2−/−; 2-tailed, unpaired Student'sttest). (c) Hepatic lactate levels of random-fed mice of indicated genotypes 7 days after transduction with HK2 adenovirus. Data are means±s.e.m.,n=3 (P<0.05 (a) versus GFP; 2-tailed, unpaired Student'sttest). (d) H&E-stained sections of WT andAlbCre;PTENf/f;Akt2−/−livers transduced with GFP or HK2 adenoviruses. Bar represents 100 μm. (e) Increased proliferation rate of hepatocytes induced by HK2 overexpression in the livers of mice of indicated genotypes. BrdU+ nuclei and total number of nuclei were scored in the livers of adenovirus-transduced mice 1 day after administration of BrdU in drinking water. Data presented as a ratio of BrdU+ to total number of nuclei ±s.e.m.,n=3–8 (P<0.05 (a) versus GFP; 2-tailed, unpaired Student'sttest). Figure 2: HK2 and PKM2 glycolytic isozyme expression promotes liver growth. ( a ) Immunoblot analysis of PKM2 and HK2 protein expression in livers of mice, 7 days after transduction with indicated adenoviruses. ( b ) Liver weight relative to body weight of mice transduced with indicated adenoviruses. Data are means±s.e.m., n =3–8 ( P <0.05 (a) versus GFP/WT; (b) versus adenoHK2/WT; (c) versus adenoPKM2/WT; (d) versus GFP/ AlbCre;PTEN f/f ;Akt2 −/− ; 2-tailed, unpaired Student's t test). ( c ) Hepatic lactate levels of random-fed mice of indicated genotypes 7 days after transduction with HK2 adenovirus. Data are means±s.e.m., n =3 ( P <0.05 (a) versus GFP; 2-tailed, unpaired Student's t test). ( d ) H&E-stained sections of WT and AlbCre;PTEN f/f ;Akt2 −/− livers transduced with GFP or HK2 adenoviruses. Bar represents 100 μm. ( e ) Increased proliferation rate of hepatocytes induced by HK2 overexpression in the livers of mice of indicated genotypes. BrdU+ nuclei and total number of nuclei were scored in the livers of adenovirus-transduced mice 1 day after administration of BrdU in drinking water. Data presented as a ratio of BrdU+ to total number of nuclei ±s.e.m., n =3–8 ( P <0.05 (a) versus GFP; 2-tailed, unpaired Student's t test). Full size image Akt2 controls PPARγ activity in PTEN -null liver Given the distinctive features of PKM2 and HK2 isozymes in regulating cell metabolism, we set out to determine the transcription factor(s) responsible for their selective Akt2-dependent regulation in PTEN -null hepatocytes. We initially considered the involvement of c-Myc and HIF1α transcription factors, two potent stimulators of glycolytic gene transcription [4] . Consistently, adenoviral transduction of c-Myc and HIF1α in primary hepatocytes increased PKM2 and HK2 expression in addition to other glycolytic enzymes such as GAPDH, PGK1, ENO1 as well as LDHA, a known non-glycolytic target of both factors ( Supplementary Fig. S4a ). However, we failed to reveal a significant regulation of c-Myc and HIF1α expression at the level of mRNA, total protein and nuclear protein in the wild type, AlbCre;PTEN f/f and AlbCre;PTEN f/f ;Akt2 −/− livers ( Supplementary Fig. S4b,c,d ). Furthermore, the HIF1α- and c-Myc-target genes GAPDH, PGK1, ENO1, were not regulated in an Akt2-dependent manner in livers ( Fig. 1 ). These observations would be consistent with extra mechanisms downstream of Akt2 controlling PKM2 and HK2 expression. We noticed that fat storing tissues also contained abundant amount of PKM2 and HK2. This was the case for the epididymal adipose tissues in wild-type mice ( Fig. 3a ), and for steatotic livers in AlbCre;PTEN f/f mice ( Fig. 1 ). PPARγ is a master regulator of adipogenesis and fat storage [21] . In liver, PPARγ levels are increased during steatosis induced by high fat diet [22] , leptin deficiency [23] , or the genetic deletion of PTEN [14] . Importantly, we found that the increase of PPARγ mRNA and nuclear protein levels in AlbCre;PTEN f/f livers was reduced by 35% and 55%, respectively, in the AlbCre;PTEN f/f ;Akt2 −/− genotype ( Fig. 3b,c ), correlating with the extent of steatosis ( Supplementary Fig. S2 ). The reduction of PPARγ expression in AlbCre;PTEN f/f ;Akt2 −/− livers was accompanied by a comparable reduction of FoXo phosphorylation ( Supplementary Fig. S5a ). FoXo transcription factor family members were previously shown to be Akt substrates and to regulate PPARγ expression in fat tissues [24] , [25] . Interestingly, Akt2 deletion also abrogated expression of hepatic Cyclooxygenase-2 ( Supplementary Fig. S5b ), a rate-limiting enzyme in prostaglandin synthesis that was previously shown to be upregulated in PTEN -null cells [26] . Although the nature of PPARγ endogenous ligands is still under debate, prostaglandins were proposed as natural regulators of PPARγ [27] . Thus, it is possible that Akt2 activity might affect both PPARγ expression and activation in liver. Consistently, Akt2 activity contributed to control of the mRNA expression of PPARγ targets, namely cluster of differentiation 36 (CD36) and cell death-inducing DFFA-like effector-C (CIDE-C) ( Fig. 3d ). Chromatin immunoprecipitation from liver extracts using PPARγ antibodies demonstrated that the binding of PPARγ to the promoter of CD36 was dependent on Akt2 activation ( Fig. 3e ). 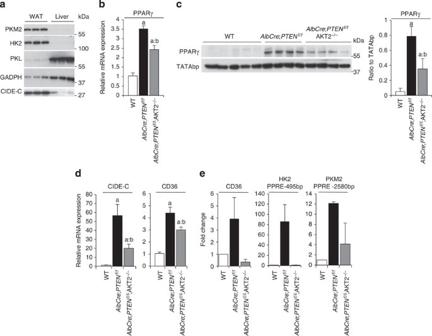Figure 3: PPARγ controls HK2 and PKM2 expression inPTEN-null liver. (a) Immunoblot analysis of protein expression in liver and WAT tissue of WT mice. (b) RT–QPCR analysis of relative transcript levels of PPARγ in the mouse livers of indicated genotypes. Data are mean ±s.e.m.,n=5 (P<0.05 (a) versus WT; (b) versusAlbCre;PTENf/f, 2-tailed, unpaired Student'sttest). (c) Immunoblot analysis showing levels of PPARγ in liver nuclear extracts. The ratio to TATA-binding nuclear protein of the densitometric assay ±s.e.m. is presented,n=4–5 (P<0.05 (a) versus WT; (b) versusAlbCre;PTENf/f, 2-tailed, unpaired Student'sttest). (d) Relative transcript levels of CD36 and CIDE-C in the mouse livers of indicated genotypes. Data are mean ±s.e.m.,n=7 (P<0.05 (a) versus WT; (b) versusAlbCre;PTENf/f; 2-tailed, unpaired Student'sttest). (e) Endogenous PPARγ chromatin immunoprecipitation assessed for CD36, PKM2 and HK2 murine promoters relative to immunoprecipitation with nonspecific IgG. Data are presented as an average of fold induction over WT control mice of two independent experiments,n=4. Figure 3: PPARγ controls HK2 and PKM2 expression in PTEN -null liver. ( a ) Immunoblot analysis of protein expression in liver and WAT tissue of WT mice. ( b ) RT–QPCR analysis of relative transcript levels of PPARγ in the mouse livers of indicated genotypes. Data are mean ±s.e.m., n =5 ( P <0.05 (a) versus WT; (b) versus AlbCre;PTEN f/f , 2-tailed, unpaired Student's t test). ( c ) Immunoblot analysis showing levels of PPARγ in liver nuclear extracts. The ratio to TATA-binding nuclear protein of the densitometric assay ±s.e.m. is presented, n =4–5 ( P <0.05 (a) versus WT; (b) versus AlbCre;PTEN f/f , 2-tailed, unpaired Student's t test). ( d ) Relative transcript levels of CD36 and CIDE-C in the mouse livers of indicated genotypes. Data are mean ±s.e.m., n =7 ( P <0.05 (a) versus WT; (b) versus AlbCre;PTEN f/f ; 2-tailed, unpaired Student's t test). ( e ) Endogenous PPARγ chromatin immunoprecipitation assessed for CD36, PKM2 and HK2 murine promoters relative to immunoprecipitation with nonspecific IgG. Data are presented as an average of fold induction over WT control mice of two independent experiments, n =4. Full size image PKM2 and HK2 are novel transcriptional targets of PPARγ By in silico analysis, it appeared that the promoter regions of PKM2 and HK2 genes also contained several PPAR response elements (PPRE). Namely, for HK2, they were localized at positions −2,694 bps, −1,216 bp, −1,162 bp, −756 bp, −495 bp and for PKM2 at −2580 bp, −2108 bp, −2086 bp, −1,927 bp, −1,028 bp and −235 bp from the transcription start site. Independent chromatin immunoprecipitation assays demonstrated that, in PTEN -deficient livers, PPARγ binding to one PPRE in the promoter of PKM2 (at −2,580 bp position) and to one PPRE in the promoter of HK2 (at −495 bp position) was enriched more than tenfold over the IgG control immunoprecipitations ( Fig. 3e ). Importantly, this binding required Akt2 activity as it was reduced in AlbCre;PTEN f/f ;Akt2 −/− livers. Taken together, these findings indicate that PKM2 and HK2 are novel and direct targets of PPARγ, consistent with their expression in adipose tissue and fatty liver. Pioglitazone treatment induces growth of PTEN -null liver Our data suggest that PPARγ may promote metabolic adaptations downstream of PI3K and Akt2 pathway favouring hepatocyte steatosis and proliferation. However, PPARγ in other systems may also promote cell differentiation and cell-cycle withdrawal [28] . Intriguingly, PTEN expression has been proposed as one of the possible mechanisms by which PPARγ may exert anti-tumoral actions [29] . Therefore, the functional outcome of PPARγ activity on PTEN -negative liver growth is difficult to predict and is important to assess, given the potential for pharmacological intervention with PPARγ synthetic ligands to treat metabolic diseases [30] . To this end, PPARγ activity was modulated in PTEN -null livers. AlbCre;PTEN f/f and wild-type mice were daily treated for 12 days with the PPARγ agonist pioglitazone. This reduced fed glycaemia in both genotypes ( Fig. 4a ), consistent with the insulin-sensitizing systemic effect of pioglitazone. However, pioglitazone promoted a 62% increase in liver/body ratio ( Fig. 4b ), and a threefold increase in BrdU-positive cells ( Fig. 4c ), exclusively in PTEN -null livers, whereas growth was not induced in wild-type liver controls in agreement with the low PPARγ expression in this genotype. Strikingly, pioglitazone selectively raised the levels of PKM2 and HK2 proteins in AlbCre;PTEN f/f livers with no effect on PKL and GAPDH levels ( Fig. 4d ). 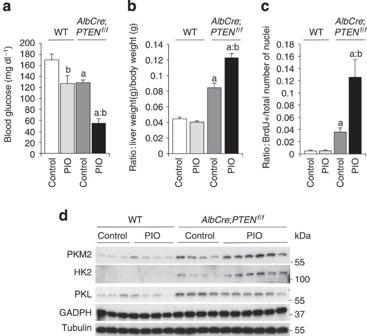Figure 4: Pharmacological activation of PPARγ by Pioglitazone promotes growth ofPTEN-null liver. (a) Blood glucose level of random-fed mice of the indicated genotypes. Data are means±s.e.m.,n=8 (P<0.05 (a) versus WT; (b) versus control; 2-tailed, unpaired Student'sttest). (b) Liver- to body-weight ratio of WT andAlbCre;PTENf/fmice after PIO treatment. Data are means±s.e.m.,n=5–8 (P<0.05 (a) versus WT; (b) versus control; 2-tailed, unpaired Student'sttest). (c) Increased proliferation rate of hepatocytes after PIO treatment. Number of BrdU+ nuclei and total number of hepatocytes nuclei were scored in the liver of untreated and PIO-treated mice, 5 days after administration of BrdU in drinking water. Data presented as a ratio of BrdU+ to total number of nuclei ±s.e.m.,n=4–8 (P<0.05 (a) versus WT; (b) versus control, 2-tailed, unpaired Student'sttest). (d) Immunoblot analysis of liver extracts of WT andAlbCre;PTENf/fmice treated with or without PIO. Figure 4: Pharmacological activation of PPARγ by Pioglitazone promotes growth of PTEN -null liver. ( a ) Blood glucose level of random-fed mice of the indicated genotypes. Data are means±s.e.m., n =8 ( P <0.05 (a) versus WT; (b) versus control; 2-tailed, unpaired Student's t test). ( b ) Liver- to body-weight ratio of WT and AlbCre;PTEN f/f mice after PIO treatment. Data are means±s.e.m., n =5–8 ( P <0.05 (a) versus WT; (b) versus control; 2-tailed, unpaired Student's t test). ( c ) Increased proliferation rate of hepatocytes after PIO treatment. Number of BrdU+ nuclei and total number of hepatocytes nuclei were scored in the liver of untreated and PIO-treated mice, 5 days after administration of BrdU in drinking water. Data presented as a ratio of BrdU+ to total number of nuclei ±s.e.m., n =4–8 ( P <0.05 (a) versus WT; (b) versus control, 2-tailed, unpaired Student's t test). ( d ) Immunoblot analysis of liver extracts of WT and AlbCre;PTEN f/f mice treated with or without PIO. Full size image PPARγ overexpression in vivo induces liver growth To analyse the effects of cell-autonomous activation of PPARγ on liver growth, wild-type, AlbCre;PTEN f/f and AlbCre;PTEN f/f ;Akt2 −/− mice were in vivo transduced with PPARγ-expressing adenoviral vector that has a pronounced tropism for liver. In line with the results of PPARγ activation by pharmacological agents, PPARγ overexpression led to a significant increase in liver/whole body ratio in wild type, AlbCre;PTEN f/f and AlbCre;PTEN f/f ;Akt2 −/− livers as compared with control transduced livers ( Supplementary Fig. S6a ). The effect on liver hypertrophy and steatosis was particularly striking in wild type and AlbCre;PTEN f/f ;Akt2 −/− tissues, that express low levels of endogenous PPARγ ( Fig. 5a ). Induction of PKM2 and HK2 by PPARγ expression was comparable to well-established PPARγ target such as CD36 ( Fig. 5b ). The massive and selective upregulation of PKM2 and HK2 over other glycolytic enzymes was confirmed at the level of both mRNA and protein ( Fig. 5b,c ). PKM1 and PKM2 isoforms are transcribed from the same PKM locus and arise from alternative splicing of PKM pre-mRNA leading to inclusion of either exon 9 in the PKM1 mature mRNA, or exon 10 in PKM2 (ref. 31 ). Despite their similarities, the effects on aerobic glycolysis and cancer progression are mainly ascribed to PKM2 rather than PKM1 (ref. 7 ). In PPARγ-transduced livers, the transcription of PKM gene was upregulated, leading to increased levels of both PKM1 and PKM2 mRNAs ( Fig. 5b ). Although the formation of both PKM splice variants was detected, PKM2 mRNA was more abundant than PKM1 ( Supplementary Fig. S6b ). Taken together, our findings indicate that PPARγ acts in vivo on PKM and HK2 gene transcription, and that hepatocytes are competent for PKM2 production. To address whether glycolysis may concur to the growth-promoting action of PPARγ in liver, PPARγ-transduced wild-type mice were treated with the glycolytic inhibitor 3-bromopyruvate (3-BrPA) [32] . 3-BrPA inhibited PPARγ-induced liver growth because of effects on hepatocyte proliferation and steatosis ( Fig. 5d,e,f ). 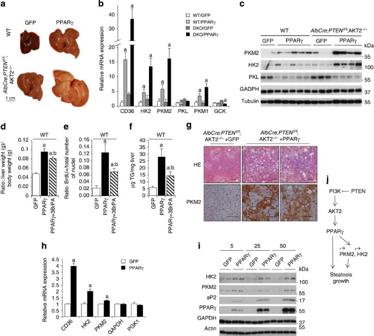Figure 5: Rescue of PPARγ expression in liver causes hypertrophy. (a) Macroscopic view of WT andAlbCre;PTENf/f;Akt2−/−mice 7 days after adenoviral transduction of GFP or PPARγ. (b) Relative transcript levels and (c) immunoblot analysis of protein levels in livers of mice transduced with GFP or PPARγ adenoviruses for 7 days. Data are means±s.e.m.,n=3–5 (P<0.05 (a) versus GFP; 2-tailed, unpaired Student'sttest). (d) Liver to body weight ratio of WT mice transduced with adenoviruses expressing GFP or PPARγ and treated with 3BrPA. Data are means±s.e.m.,n=5–11 (P<0.05 (a) versus WT; (b) versus PPARγ control; 2-tailed, unpaired Student'sttest). (e) Hepatocyte proliferation after PPARγ overexpression is inhibited by 3BrPA treatment. Number of BrdU+ nuclei and total number of hepatocyte nuclei were scored in the livers of mice transduced with indicated adenoviruses treated for 1 day before sacrifice with BrdU in drinking water. Data are presented as a ratio of BrdU+ to total number of nuclei ±s.e.m.,n=3–7 (P<0.05 (a) versus GFP; (b) versus PPARγ control; 2-tailed, unpaired Student'sttest). (f) Triglyceride concentration in liver tissue of mice transduced with GFP or PPARγ adenoviruses, and treated with 3BrPA. Data are means±s.e.m.,n=5–11 (P<0.05 (a) versus GFP; (b) versus PPARγ control; 2-tailed, unpaired Student'sttest). (g) H&E staining and immunohistochemistry using anti-PKM2 antibody of liver sections ofAlbCre;PTENf/f;Akt2−/−mice 14 days after adenoviral transduction with GFP or PPARγ. Bar represents 100 μm. (h) RT–QPCR analysis of relative transcript levels of glycolytic enzymes in primary WT hepatocytes 40 h postinfection with 5 MOI of adenoviruses expressing GFP or PPARγ. Data are means±s.e.m.,n=3 (P<0.05 (a) versus GFP; 2-tailed, unpaired Student'sttest). (i) Immunoblot analysis of protein levels of glycolytic enzymes in primary hepatocytes transduced with different doses of PPARγ or GFP adenovirus collected 40 h postinfection. (j) Proposed model of PPARγ contribution to metabolic changes and pathophysiological growth inPTEN-null livers. Figure 5: Rescue of PPARγ expression in liver causes hypertrophy. ( a ) Macroscopic view of WT and AlbCre;PTEN f/f ;Akt2 −/− mice 7 days after adenoviral transduction of GFP or PPARγ. ( b ) Relative transcript levels and ( c ) immunoblot analysis of protein levels in livers of mice transduced with GFP or PPARγ adenoviruses for 7 days. Data are means±s.e.m., n =3–5 ( P <0.05 (a) versus GFP; 2-tailed, unpaired Student's t test). ( d ) Liver to body weight ratio of WT mice transduced with adenoviruses expressing GFP or PPARγ and treated with 3BrPA. Data are means±s.e.m., n =5–11 ( P <0.05 (a) versus WT; (b) versus PPARγ control; 2-tailed, unpaired Student's t test). ( e ) Hepatocyte proliferation after PPARγ overexpression is inhibited by 3BrPA treatment. Number of BrdU+ nuclei and total number of hepatocyte nuclei were scored in the livers of mice transduced with indicated adenoviruses treated for 1 day before sacrifice with BrdU in drinking water. Data are presented as a ratio of BrdU+ to total number of nuclei ±s.e.m., n =3–7 ( P <0.05 (a) versus GFP; (b) versus PPARγ control; 2-tailed, unpaired Student's t test). ( f ) Triglyceride concentration in liver tissue of mice transduced with GFP or PPARγ adenoviruses, and treated with 3BrPA. Data are means±s.e.m., n =5–11 ( P <0.05 (a) versus GFP; (b) versus PPARγ control; 2-tailed, unpaired Student's t test). ( g ) H&E staining and immunohistochemistry using anti-PKM2 antibody of liver sections of AlbCre;PTEN f/f ;Akt2 −/− mice 14 days after adenoviral transduction with GFP or PPARγ. Bar represents 100 μm. ( h ) RT–QPCR analysis of relative transcript levels of glycolytic enzymes in primary WT hepatocytes 40 h postinfection with 5 MOI of adenoviruses expressing GFP or PPARγ. Data are means±s.e.m., n =3 ( P <0.05 (a) versus GFP; 2-tailed, unpaired Student's t test). ( i ) Immunoblot analysis of protein levels of glycolytic enzymes in primary hepatocytes transduced with different doses of PPARγ or GFP adenovirus collected 40 h postinfection. ( j ) Proposed model of PPARγ contribution to metabolic changes and pathophysiological growth in PTEN -null livers. Full size image The liver-cell type expressing PKM2 after PPARγ expression was determined by immunostaining as the hepatocytes ( Fig. 5g ), ruling out the contribution of other cell types to the observed effects on PKM2 expression. It was also independently confirmed by modulating PPARγ levels in primary hepatocyte cultures by adenoviral transduction, where increasing doses of PPARγ upregulated HK2 and PKM2 mRNA and protein levels ( Fig. 5h and i ). PPARγ overexpression had similar effects on the well-established targets CD36 and aP2, whereas the levels of other glycolytic enzymes such as GAPDH and PGK1 remained constant. Conversely, overexpression of PPARα was not able to stimulate HK2 and PKM2 mRNA levels in primary hepatocytes ( Supplementary Fig. S7a ). Moreover, PPARα and PPARβ expression was not regulated by Akt2 in livers ( Supplementary Fig. S7b ). Altogether, our data suggest a cell-autonomous regulation of HK2 and PKM2 specifically by the γ type of PPARs. Strikingly, the AlbCre;PTEN f/f ;Akt2 −/− livers showed pathological signs 2 weeks after adeno-PPARγ transduction, including bile duct hyperplasia, hepatic lobule disorganization, and ballooning hepatocytes ( Fig. 5g ). Thus, PPARγ orchestrates a gene-expression program downstream the PI3K/Akt2 pathway, favouring aerobic glycolysis, lipogenesis and pathophysiological growth. Although the role of c-Myc and HIF-1α in general regulation of glycolytic enzyme expression is well documented, our understanding of molecular mechanisms selectively controlling specific glycolytic enzymes is limited. Regulation of HK2 and PKM2 isozymes is especially interesting, owing to their function in aerobic glycolysis and growth. Here we provide evidence that PPARγ has an important role in HK2 and PKM2 glycolytic isozyme gene trascription in PTEN -null fatty liver. We propose that these novel targets, in addition to other well-established target genes, concur to the growth and metabolic adaptation of liver to nutrition, insulin, PI3K, Akt2 and PPARγ signalling: aerobic glycolysis, steatosis and hepatomegaly ( Fig. 5j ). Intense efforts have been made to evaluate whether therapy with insulin-sensitizing agents, and PPARγ agonists could be beneficial against steatosis-associated human liver diseases, though the outcome is not conclusive yet [30] . The rationale behind these clinical trials is that PPARγ agonists should alleviate liver steatosis, promoting lipid accumulation in adipose tissue and suppressing hepatic inflammation. This strategy may be appropriate when the origin of liver steatosis is environmental, owing to nutritional habits. However, liver steatosis and hepatic PPARγ expression may arise from genetic insults, as observed when PTEN is deleted and Akt2 upregulated in hepatocytes. In these cases, we show that PPARγ activation is detrimental, leading to massive steatosis and hepatocyte proliferation. Regulation of HK2 and PKM2 by hepatic PPARγ is observed well before tumour onset, which in PTEN -deficient livers appears since 7 months of age. It is tempting to speculate that these effects may be causally involved in the well-established correlation between liver steatosis and increased cancer risk. Whereas PPARγ may act as a tumour suppressor in colon, breast and prostate cancers [33] , [34] , PPARγ activation promotes polyp formation in colon cells carrying mutations in the APC gene [35] , [36] , [37] . Interestingly, in liver, histone deacetylase 3 (Hdac3) and nuclear hormone co-repressor (N-CoR) are recruited by several nuclear hormone receptors, including PPARγ, to regulate transcription in the absence of the ligand. Loss-of-function mutations in these transcriptional repressors promote steatosis and pathological liver growth culminating in cancer in mice and humans [38] , [39] . These studies in combination with our data suggest a functional PPARγ/Hdac3/N-CoR complex in the regulation of liver metabolism, which may have important implications in tumorigenesis. Animal experiments Generation of AlbCre;PTEN f/f and Akt2 −/− mice has been previously described [14] , [16] . Mice were maintained at 22 °C with a 12-h-dark/12-h-light cycle and had free access to food. All animal studies were approved by the Direction Départementale des Services Vétérinaires, Préfecture de Police, Paris, France (authorization number 75-1313). Pioglitazone was diluted in 0.5% carboxymethyl cellulose and was administered at 30 mg kg −1 dose by daily gavage for 12 days. Group of wild-type mice transduced with PPARγ adenovirus were treated with 4 mg kg −1 3-BrPA (Sigma) freshly prepared in PBS and adjusted to pH7.4. The drug was injected intraperitoneally every day for 7 days. The first injection was 12 h after transduction with adenovirus. Adenoviruses Recombinant adenovirus expressing untagged full-length human PPARγ2 was a generous gift from Renaud Dentin (Institut Cochin, INSERM U1016, UMR8104). Recombinant adenovirus expressing c-Myc was a generous gift from Heiko Hermeking (Institute of Pathology Ludwig-Maximilians-University Munich) [40] . Recombinant adenovirus expressing HIF-1αCA5 mutant was a generous gift from Gregg L. Semenza (The Johns Hopkins University School of Medicine) [41] . Recombinant adenovirus expressing untagged full-length mouse PPARα was described previously [42] . Recombinant adenovirus expressing V5-tagged full-length human HK2 was custom-generated at GeneCust. Recombinant adenovirus expressing untagged human PKM2 was acquired from Excellgen. Viruses were generated through homologous recombination between a linearized transfer vector pAD-Track and the adenoviral backbone vector pAD-Easy. Viruses were purified by the CsCl method and dialysed against PBS buffer containing 7% glycerol. For in vivo transduction, 10 9 of adenoviral infectious particles were diluted in 0.9%NaCl and administered retro-orbitally, using 26G needle in total volume of 100 μl per mouse, and mice were killed 7 or 14 days postinfection. Adenovirus coding for GFP was used as a control in all experiments. Metabolic studies in mice At 3 months of age, a glucose tolerance test was performed in mice after an overnight fasting (14 h). Mice were intraperitoneally injected with 2 g kg −1 glucose, and blood was collected from the tail vein for determination of glucose levels at 0, 15, 30, 45 and 100 min by Glucotrend glucometer (Roche Diagnostics). Insulin tolerance test was performed at 3 months of age. Overnight-fasted mice were intraperitoneally injected with 1 U kg −1 insulin (Actrapid), and the glucose concentration in whole blood from the tail vein was measured at 0, 15, 30 and 60 min. Fasting insulin levels were measured by ELISA assay (Crystal chem). Immunohistochemistry and morphometric analysis Liver tissue was fixed overnight in phosphate-buffered 10% formalin and embedded in paraffin, sectioned in 4 μm, and stained with eosin/hematoxylin. Immunohistochemistry was performed using anti-BrdU antibody (Roche), anti-β-catenin (Calbiochem) and anti-PKM2xp (Cell Signalling Technology) antibodies. For 5-bromo-2′deoxyuridine (BrdU) incorporation, mice were fed with BrdU (3 mg ml −1 , Sigma-Aldrich) dissolved in drinking water for either for 5 days (PIO treatment) or last 24 h (adenoviral transduction) before killed. The results were expressed as the ratio of BrdU-positive nuclei and total number of nuclei in at least 10 areas of 33,500 μm 2 for anti-BrdU staining analysed. Subcellular fractionation and western blot Mitochondria were isolated as previously described [43] . Briefly, 50–100 mg of snap-frozen liver tissue was homogenized in IBc buffer complemented with complete protease inhibitors (Roche). After centrifugation at 600 g for 10 min, the supernatant containing the mitochondria was centrifugated at 7,000g for 10 min. The pellet of mitochondria was washed three times with IBc buffer and, after the final centrifugation, the mitochondria were lysed in extraction buffer (20 mM Tris–HCl (pH 8,0), 5% glycerol, 138 mM NaCl, 2,7 mM KCl, 1% NP-40, 20 mM NaF, 5 mM EDTA, 1 mM DTT) complemented with complete protease inhibitors (Roche). Nuclear extracts were prepared using NE-PER Kit (Pierce), according to manufacturer's recommendations, using 50–100 mg of snap-frozen liver tissue as a starting material. Total protein extracts were prepared as described before [44] . Proteins were resolved by SDS–PAGE, transferred to polyvinylidene difluoride membrane and incubated with anti-phospho Akt (Ser473), anti-aP2, anti-PKM2, anti-HK2, anti-Akt, anti-c-Myc, anti-Lamin A/C, anti-phosphoFoXo1/3a (Thr24/32), anti-FoXo3a, anti-phosphoGSK3β (Ser9), anti-GSK3β (Cell Signalling), anti-PKL (a generous gift of Benoit Viollet, Cochin Institut, Paris), anti-tubulin and anti-β-actin (Sigma), anti-VDAC and anti-CIDE-C (Millipore), anti-HK2, anti-TATABP, anti-PPARγ and anti-enolase (Santa Cruz), anti-GAPDH and anti-V5 (Abcam), anti-HIF1α (Novus) antibodies. Hepatic metabolites analysis TG levels were determined using Triglycerides FS Kit (Diasys) according to the manufacturer's instructions. 50–100 mg of powdered liver tissue or pelleted primary hepatocytes were used for acetone extraction. Lactate concentrations were assayed in liver extracts of random-fed mice as described previously [45] . Briefly, metabolites were extracted in 9% perchloric acid from clamp-frozen liver tissues, neutralized using potassium hydroxide, and assayed using a spectrophotometric enzymatic procedure. Lactate levels after adenovirus-mediated HK2 overexpression were determined using Lactate reagent (Trinity Biotech) using 50–100 mg of liver tissue or cell culture medium supernatants. Liver tissue extracts before measurement were filtered using 10 K Amicon Ultra columns (Millipore). RT–QPCR Total RNA was isolated from 50–100 mg of snap-frozen liver tissue using a RNAeasy Lipid Tissue Midi or Mini Kit (Qiagen). Total RNA from hepatocytes was isolated using a RNAeasy Mini Kit (Qiagen). Single-strand complementary DNA was synthesized from 1 μg of total RNA with random hexamer primers and SuperScript II (Invitrogen). Real-time quantitative PCR (RT–QPCR) was performed on Taqman instrument (Applied Biosystem) using a SYBR Green PCR Master Mix (Applied Biosystem). The relative amounts of the mRNAs studied were determined by means of the 2 −ΔΔCT method, with pinin, actin or cyclophilin as reference genes and control-treated samples as the invariant controls. Primers used for analysis are listed in Supplementary Table S1 . For PKM isoform ratio analysis, 1 microlitre of the complementary DNA was amplified using DreamTaq Green PCR Master Mix (Fermentas) in total volume of 50 microlitres. Five microlitres of PCR product was digested by FastDigest EcoNI (Fermentas) and the products analysed on agarose gel. An EcoNI site is present in exon 9 of mouse PKM1, whereas it is absent in exon 10 of PKM2. Primers used for amplification of PKM isoform identification are shown in Supplementary Table S2 . Chromatin immunoprecipitation Random-fed mice were used for experiment with two mice of the same genotype used for preparation in each sample for each independent experiment. Chromatin was prepared from freshly dissected liver, as previously described [46] , [47] . Chromatin was sonicated in SBAR buffer (50 mM HEPES, 140 mM NaCl, 1 mM EDTA, 1% Triton, 0.1% sodium deoxycholate and 0.1% SDS with complete protease inhibitors (Roche) and incubated with antibody to PPARγ (Santa Cruz, sc-7196) or IgG as control. Next, immunocomplexes were recovered with Protein A sepharose beads (Amersham). After washing, DNA–protein complexes were eluted and cross-linking was reversed by heating the samples at 65 °C for 16 h. DNA was then purified using Qiagen PCR purification kit. Real-time quantitative PCR (RT–QPCR) was performed using a Taqman instrument (Applied Biosystem) according to the manufacturer's instructions, using a SYBR Green PCR Master Mix (Applied Biosystem). The relative amounts of the immunoprecipitated DNA were determined by means of the 2 −ΔCT method, with input DNA values for each sample as the control. The enrichment over IgG control of more than tenfold was considered as a cutoff. The results are presented as average of fold induction over wild type (WT) for the PPREs confirmed in independent experiments. The location of putative PPREs within promoter region of PKM2 and HK2 genes was determined using MatInspector software (Genomatix) and 3 kb fragment of DNA sequence upstream the transcription start. Numerous potential PPREs were located upstream first exon of HK2 and PKM2 genes: HK2: −2,694 bp; −1,216 bp; −1,162 bp; −756 bp; −495 bp; PKM2: −2,580 bp; −2,108 bp; −2,086 bp; −1,927 bp; −1,028 bp; −235 bp. Confirmed PPREs for PKM2 and HK2 promoters are PKM2: −2,580 bp; HK2: −495 bp. The primer pairs flanking putative PPREs used for amplification have been designed using PrimerBlast software and are listed in Supplementary Table S3 . Hepatocyte culture Primary hepatocytes were isolated from wild-type C57BL/6J mice by collagenase perfusion method as described previously [44] . 4×10 5 cells were plated in 6-well plates in William's medium (Invitrogen) supplemented by 20% FBS, INS (4 μg ml −1 ), 10 units ml −1 penicillin, 10 g ml −1 streptomycin, and 25 nM dexamethasone (Sigma). After attachment, cells were transduced with adenoviruses expressing GFP, PPARα, PPARγ2, c-Myc or HIF-1αCA5 in serum-free William's medium for 2 h in 5-50 MOI dose as indicated. Subsequently, medium was changed and cells were maintained in serum-free William's medium complemented with INS and dexametasone. How to cite this article: Panasyuk, G. et al . PPARγ contributes to PKM2 and HK2 expression in fatty liver. Nat. Commun. 3:672 doi: 10.1038/ncomms1667 (2012).